SHP-1-mediated inhibitory signals promote responsiveness and anti-tumour functions of natural killer cells Natural killer (NK) cells are cytotoxic innate lymphoid cells that are involved in immune defense. NK cell reactivity is controlled in part by MHC class I recognition by inhibitory receptors, but the underlying molecular mechanisms remain undefined. Using a mouse model of conditional deletion in NK cells, we show here that the protein tyrosine phosphatase SHP-1 is essential for the inhibitory function of NK cell MHC class I receptors. In the absence of SHP-1, NK cells are hyporesponsive to tumour cells in vitro and their early Ca 2+ signals are compromised. Mice without SHP-1 in NK cells are unable to reject MHC class I-deficient transplants and to control tumours in vivo . Thus, the inhibitory activity of SHP-1 is needed for setting the threshold of NK cell reactivity. Natural killer (NK) cells are cytotoxic innate lymphoid cells (ILCs) that produce various chemokines and cytokines, including interferon-γ (IFN-γ) [1] , [2] , [3] . NK cells are involved in the immune surveillance of tumours and microbes, such as viruses, fungi, intracytoplasmic bacteria and parasites [4] , [5] , [6] . Despite their classification as innate lymphocytes, it is becoming clear that NK cells also have adaptive features, including some memory properties in particular [7] , [8] . NK cells identify their targets via a panel of cell surface receptors, including inhibitory receptors, adhesion molecules and activating receptors recognizing microbe-derived molecules and stress-induced self-derived molecules [2] . The inhibitory NK cell surface receptors interacting with major histocompatibility complex (MHC) class I molecules are the best characterized, and have been shown to contribute to host tolerance of NK cells [9] , [10] , [11] . When NK cells interact with cells expressing surface MHC class I, the engagement of their cognate inhibitory receptors induces inhibitory signals that limit NK cell activation. By contrast, when NK cells interact with cells with a low density of surface MHC class I, the lack of engagement of MHC class I-specific inhibitory receptors promotes NK cell activation. Consequently, NK cells can eliminate MHC class I-negative cells [12] , [13] . However, no signs of NK cell-dependent autoimmunity have been detected in mice or humans with genetic defects, resulting in a lack of stable cell surface expression of MHC class I molecules [14] . In these MHC class I-deficient hosts, NK cells are present but hyporesponsive to various stimuli, providing a basis for self-tolerance. This situation is not limited to MHC class I-deficient hosts, as subsets of NK cells lacking inhibitory cell surface receptors recognizing host MHC class I molecules are present in normal humans and mice [14] . Paradoxically, the sustained lack of engagement of inhibitory receptors is thus involved in establishing the hyporesponsiveness of NK cells observed in MHC class I-deficient hosts [15] , [16] , [17] , [18] . Nevertheless, the precise mechanisms by which the inhibitory receptors exert their effects on the acquisition or maintenance of NK cell functional competence, referred to as NK cell education or tuning, remain a matter of debate. It has been suggested that the recognition of MHC class I molecules by inhibitory receptors licences NK cells to acquire their effector functions, in a process referred to as arming [19] . Alternatively, it has been suggested that NK cells integrate activating signals that desensitize them, leading to their hyporesponsiveness, unless this effect is attenuated by the binding of inhibitory receptors to their MHC class I ligands, in a process referred to as disarming [14] . In both cases, the impact of MHC class I receptors on NK cell responsiveness does not follow an all-or-none law, instead following a rheostat model, in which NK cell reactivity increases quantitatively with each inhibitory receptor binding to self MHC class I molecules [10] , [20] . NK cell inhibitory MHC class I receptors include killer cell Ig-like receptors (KIR) in humans, inhibitory Ly49 receptors in the mouse and inhibitory CD94/NKG2A heterodimers in both species. All these inhibitory receptors harbour intracytoplasmic immunoreceptor tyrosine-based inhibition motifs (ITIMs), which are involved in their inhibitory function [21] , [22] . Following binding to MHC class I ligands, ITIMs undergo tyrosine phosphorylation, enabling them to recruit the protein tyrosine phosphatases SHP-1 and SHP-2 (refs 21 , 22 ). It has been suggested that inhibitory KIR function also involves phosphorylation of the Crk adaptor [23] , [24] . In mice, intact ITIMs are required for the function of MHC class I receptors in NK cell education [15] , [25] , [26] , but the reported role of SHP-1 remains controversial. Studies of SHP-1-deficient mice with chimeric bone marrow have shown SHP-1 to be dispensable for NK cell education [15] , whereas a transdominant negative form of SHP-1 was found to affect NK cell responsiveness [27] . However, SHP-1 is broadly expressed in haematopoietic cells, and the exploration of NK cell development and function in the absence of SHP-1 is hampered by the major inflammatory conditions prevailing in the two mouse models of SHP-1-deficiency: motheaten (Ptpn6 me/me ) and motheaten-viable (Ptpn6 me-v/me-v ) mice. Both these models display a complex inflammatory phenotype, including sterile pneumonia, dermatitis and autoimmunity, leading to premature death [28] . It is thus difficult to discriminate between the direct and indirect defects of an absence of SHP-1 on NK cells. We addressed this question, by creating a model of conditional Ptpn6 deletion, to dissect the role of SHP-1 in NK cells and the mechanisms by which the inhibitory Ly49 and CD94/NKG2A receptors affect NK cells. We found that in the absence of SHP-1, NK cells are hyporesponsive in vitro and in vivo . We also show that SHP-1 is a major mediator of the inhibitory function of MHC class I-specific receptors. Thus, SHP-1 governs the tuning of NK cells, and the inhibitory function of MHC class I-specific receptors is associated with their role in NK cell education. Deletion of SHP-1 in NK cells We used Ncr1 iCre/+ mice [29] to eliminate SHP-1 selectively from NK cells and NKp46 + ILCs (also called NCR + ILC3) by crossing with knock-in mice in which the first nine exons of the gene encoding SHP-1 ( Ptpn6 ) had been floxed [30] ( Supplementary Fig. 1 ). Unlike motheaten mice, which present a phenotype of massive inflammation leading to premature death, Ncr1 iCre/+ Ptpn6 flx/flx mice were obtained at Mendelian frequencies; they developed normally and were fertile. No statistically significant differences in the numbers and percentages of cells of the lymphoid and myeloid subsets were detected by flow cytometry analyses of the blood, spleen and liver cells from Ncr1 iCre/+ Ptpn6 +/+ mice and Ncr1 iCre/+ Ptpn6 flx/flx mice ( Fig. 1a and Supplementary Fig. 2 ). In particular, splenic CD3 − NKp46 + NK cell counts were 3.5±1.2 × 10 6 (mean±s.d., n =16) in Ncr1 iCre/+ Ptpn6 +/+ mice and 3.6±1.4 × 10 6 in Ncr1 iCre/+ Ptpn6 flx/flx mice ( Fig. 1a ). NK cell and NCR + ILC3 cell numbers were also normal in the small intestine of Ncr1 iCre/+ Ptpn6 flx/ flx mice ( Fig. 1b ), and CD49a − CD49b + NK cells and tissue-resident CD49a + CD49b − NK cells were present in normal numbers in the liver ( Fig. 1c ). The presence of NK cells in Ncr1 iCre/+ Ptpn6 flx/flx mice made it possible for us to check that SHP-1 was depleted selectively from NK cells and not from other splenocytes. In Ncr1 iCre/+ Ptpn6 flx/flx mice, the SHP-1 protein was indeed undetectable in NK cells, but was present in other splenocytes ( Fig. 1d and Supplementary Fig. 3 ), consistent with both the specificity of Ncr1 iCre/+ targeting [29] and the efficacy of SHP-1 ablation observed in B cells [32] , T cells [33] , dendritic cells and neutrophils [34] when Ptpn6 flx/flx mice were crossed with other Cre knock-in mice. The elimination of SHP-1 from NKp46 + cells therefore led to no gross abnormalities in the development of these cells and no massive inflammatory disease was observed in Ncr1 iCre/+ Ptpn6 flx/flx mice. This made it possible to carry out an unprecedented dissection of the functional consequences of an absence of SHP-1 in NK cells. 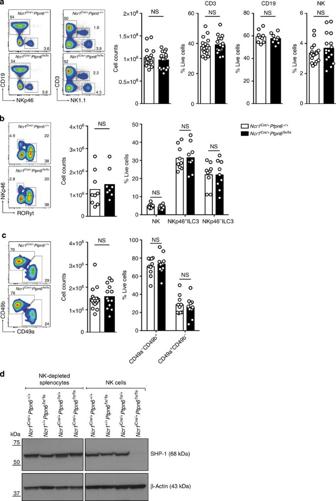Figure 1: Deletion of SHP-1 in NK cells. (a) Left panels: representative cytometric profiles of splenocytes fromNcr1iCre/+Ptpn6+/+andNcr1iCre/+Ptpn6flx/flxmice stained with anti-CD19, anti-NKp46, anti-CD3 and anti-NK1.1 mAbs. Right panels: histograms show total splenic lymphocyte counts (n=17,P=0.7554), percentages of CD3+T cells (n=17,P=0.5570), CD19+B cells (n=9,P=0.5346) and CD3−NK1.1+NK cells (n=17,P=0.3046). Statistics were performed using a Mann–Whitney test. (b) Left panels: representative cytometric profiles of CD3−gut lymphocytes fromNcr1iCre/+Ptpn6+/+andNcr1iCre/+Ptpn6flx/flxmice stained with anti-NKp46 and anti-RORγt mAbs. Right panels: histograms show total gut lymphocyte counts (n=9,P=0.2864, Mann–Whitney) and percentages of NK (CD3−NKp46+RORγt+), NKp46−ILC3 (CD3−NKp46−RORγt+) and NKp46+ILC3 (CD3−NKp46+RORγt+) cells (n=9,P>0.9999, two-way analysis of variance (ANOVA) with Bonferroni correction). (c) Left panels: representative cytometric profiles of liver lymphocytes fromNcr1iCre/+Ptpn6+/+andNcr1iCre/+Ptpn6flx/flxmice stained with anti-CD49a and anti-CD49b mAbs. Right panels: histograms show total liver lymphocyte counts (n=15,P=0.6118, Mann–Whitney) and percentages of liver CD49a−CD49b+and CD49a+CD49b−cells (n=10,P>0.9999, two-way ANOVA with Bonferroni correction). Each dot on the histograms corresponds to the data for a single mouse. The data show the results of at least four independent experiments. (d) Analysis of SHP-1 protein expression by immunoblotting in NK-depleted splenocytes (left panel) and LAK cells (right panel) prepared from the indicated mice. Representative of three independent experiments. Figure 1: Deletion of SHP-1 in NK cells. ( a ) Left panels: representative cytometric profiles of splenocytes from Ncr1 iCre/+ Ptpn6 +/+ and Ncr1 iCre/+ Ptpn6 flx/flx mice stained with anti-CD19, anti-NKp46, anti-CD3 and anti-NK1.1 mAbs. Right panels: histograms show total splenic lymphocyte counts ( n =17, P =0.7554), percentages of CD3 + T cells ( n =17, P =0.5570), CD19 + B cells ( n =9, P =0.5346) and CD3 − NK1.1 + NK cells ( n =17, P =0.3046). Statistics were performed using a Mann–Whitney test. ( b ) Left panels: representative cytometric profiles of CD3 − gut lymphocytes from Ncr1 iCre/+ Ptpn6 +/+ and Ncr1 iCre/+ Ptpn6 flx/flx mice stained with anti-NKp46 and anti-RORγt mAbs. Right panels: histograms show total gut lymphocyte counts ( n =9, P =0.2864, Mann–Whitney) and percentages of NK (CD3 − NKp46 + RORγt + ), NKp46 − ILC3 (CD3 − NKp46 − RORγt + ) and NKp46 + ILC3 (CD3 − NKp46 + RORγt + ) cells ( n =9, P >0.9999, two-way analysis of variance (ANOVA) with Bonferroni correction). ( c ) Left panels: representative cytometric profiles of liver lymphocytes from Ncr1 iCre/+ Ptpn6 +/+ and Ncr1 iCre/+ Ptpn6 flx/flx mice stained with anti-CD49a and anti-CD49b mAbs. Right panels: histograms show total liver lymphocyte counts ( n =15, P =0.6118, Mann–Whitney) and percentages of liver CD49a − CD49b + and CD49a + CD49b − cells ( n =10, P >0.9999, two-way ANOVA with Bonferroni correction). Each dot on the histograms corresponds to the data for a single mouse. The data show the results of at least four independent experiments. ( d ) Analysis of SHP-1 protein expression by immunoblotting in NK-depleted splenocytes (left panel) and LAK cells (right panel) prepared from the indicated mice. Representative of three independent experiments. Full size image Changes to NK cell surface phenotype in absence of SHP-1 We investigated the impact of a lack of SHP-1 on the various stages of NK cell maturation. The absence of SHP-1 from NK cells resulted in moderate changes to the maturation profile of these cells, as shown by the higher proportion of CD11b + CD27 + NK cells and the corresponding lower proportion of CD11b + CD27 − cells in Ncr1 iCre/+ Ptpn6 flx/flx mice than in Ncr1 iCre/+ Ptpn6 +/+ control mice ( Fig. 2a ). The KLRG1 + splenic NK cell subset population was much smaller in Ncr1 iCre/+ Ptpn6 flx/flx mice than in control mice ( Fig. 2b ). KLRG1 is a cell surface receptor, the extracytoplasmic domain of which interacts with cadherins, whereas the intracytoplasmic ITIM recruits the SHIP-1 inositol phosphatase [31] . The biological relevance of KLRG1 expression on NK cells in vivo remains unclear [32] , but KLRG1 is preferentially expressed on mature CD11b + CD27 − NK cells [33] . The lower proportion of CD11b + CD27 − cells in Ncr1 iCre/+ Ptpn6 flx/flx mice could not account for the weaker KLRG-1 expression in these mice, as the fraction of KLRG-1 + cells among CD11b + CD27 − NK cells was also lower ( Supplementary Fig. 4 ). Similar observations were made for NK cells isolated from the liver ( Supplementary Fig. 5 ), highlighting the impact of SHP-1 on KLRG1 expression. A similar decrease in the size of the KLRG1 + NK cell subset regardless of CD11bCD27 maturation phenotype has been consistently observed in MHC class I-deficient mice [34] ( Supplementary Fig. 6 ). 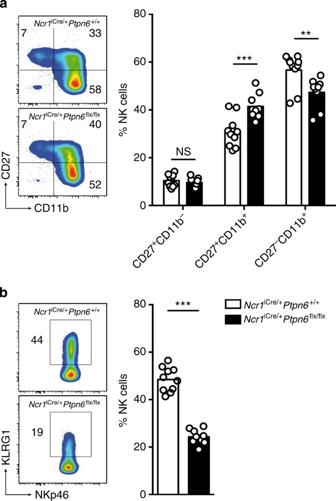Figure 2: Alteration of NK cell surface phenotype in the absence of SHP-1. (a) Left panel: representative cytometric profiles of splenic NK cells stained with anti-CD27 and anti-CD11b mAbs. Right panel: histograms show the percentages of CD27+CD11b−(P>0.9999), CD27+CD11b+(P=0.0002) and CD27−CD11b+(P=0.0011) NK cells. (n=10, two-way analysis of variance with Bonferroni correction). (b) Left panel: representative cytometric profiles of splenic NK cells stained with anti-KLRG1 and anti-NKp46 mAbs. Right panel: histograms show the percentages of KLRG1+NK cells fromNcr1iCre/+Ptpn6+/+andNcr1iCre/+Ptpn6flx/flxmice (n=10,P<0.0001, Mann–Whitney). Each dot on the histograms corresponds to the data for a single mouse and the data show the results of four independent experiments. Figure 2: Alteration of NK cell surface phenotype in the absence of SHP-1. ( a ) Left panel: representative cytometric profiles of splenic NK cells stained with anti-CD27 and anti-CD11b mAbs. Right panel: histograms show the percentages of CD27 + CD11b − ( P >0.9999), CD27 + CD11b + ( P =0.0002) and CD27 − CD11b + ( P =0.0011) NK cells. ( n =10, two-way analysis of variance with Bonferroni correction). ( b ) Left panel: representative cytometric profiles of splenic NK cells stained with anti-KLRG1 and anti-NKp46 mAbs. Right panel: histograms show the percentages of KLRG1 + NK cells from Ncr1 iCre/+ Ptpn6 +/+ and Ncr1 iCre/+ Ptpn6 flx/flx mice ( n =10, P <0.0001, Mann–Whitney). Each dot on the histograms corresponds to the data for a single mouse and the data show the results of four independent experiments. Full size image Skewing of Ly49 receptor repertoire in the absence of SHP-1 The absence of SHP-1 in NK cells had a marked effect on the expression of inhibitory Ly49 receptors. The NK cell subsets expressing Ly49A, Ly49C/I, Ly49F or Ly49G2 were larger in Ncr1 iCre/+ Ptpn6 flx/flx mice than in Ncr1 iCre/+ Ptpn6 +/+ control mice ( Fig. 3a ). This effect was specific to the inhibitory Ly49 receptors, as no change in the expression of the activating Ly49D and Ly49H receptors, NKG2A or NKG2D, was observed in the absence of SHP-1 ( Fig. 3b ). Similarly, the repertoire of inhibitory Ly49 receptors, but not of activating Ly49 receptors, is altered in MHC class I-deficient mice [35] , [36] ( Supplementary Fig. 7a,b ). Thus, two major features of NK cells in MHC class I-deficient mice—low levels of KLRG1 expression and high levels of expression of the inhibitory Ly49 receptors—were found in Ncr1 iCre/+ Ptpn6 flx/flx mice. 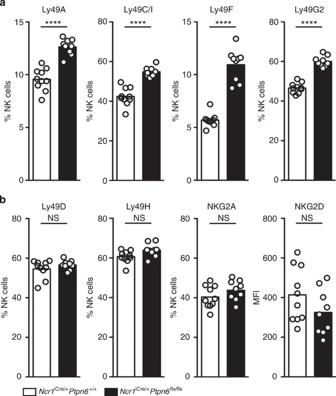Figure 3: Skewing of Ly49 receptor repertoire in the absence of SHP-1. (a) Percentages of NK cells expressing cell surface Ly49 inhibitory receptors (Ly49A, Ly49C/I, Ly49F and Ly49G2) inNcr1iCre/+Ptpn6+/+andNcr1iCre/+Ptpn6flx/flxNK cells. (n=10,P<0.0001, Mann–Whitney). (b) Percentages of NK cells expressing cell surface the NKG2A (P=0.1894) inhibitory receptor or Ly49 activating receptors (Ly49D,P=0.5633 and Ly49H,P=0.0683) and mean fluorescence intensity (MFI) of NKG2D (P=0.1752) inNcr1iCre/+Ptpn6+/+andNcr1iCre/+Ptpn6flx/flxNK cells. (n=10, Mann–Whitney). Each dot on the histograms corresponds to the data from a single mouse and the data show the results of four independent experiments. Figure 3: Skewing of Ly49 receptor repertoire in the absence of SHP-1. ( a ) Percentages of NK cells expressing cell surface Ly49 inhibitory receptors (Ly49A, Ly49C/I, Ly49F and Ly49G2) in Ncr1 iCre/+ Ptpn6 +/+ and Ncr1 iCre/+ Ptpn6 flx/flx NK cells. ( n =10, P <0.0001, Mann–Whitney). ( b ) Percentages of NK cells expressing cell surface the NKG2A ( P =0.1894) inhibitory receptor or Ly49 activating receptors (Ly49D, P =0.5633 and Ly49H, P =0.0683) and mean fluorescence intensity (MFI) of NKG2D ( P =0.1752) in Ncr1 iCre/+ Ptpn6 +/+ and Ncr1 iCre/+ Ptpn6 flx/flx NK cells. ( n =10, Mann–Whitney). Each dot on the histograms corresponds to the data from a single mouse and the data show the results of four independent experiments. Full size image In vitro NK cell hyporesponsiveness in the absence of SHP-1 We then investigated the reactivity of NK cells in Ncr1 iCre/+ Ptpn6 flx/flx mice, comparing it with that of NK cells from Ncr1 iCre/+ Ptpn6 +/+ mice. Splenic NK cells were cultured in vitro with interleukin (IL)-2 to generate lymphocyte-activated killer (LAK) cells. The proliferative response of NK cells to IL-2 was unaffected by the absence of SHP-1 ( Fig. 4a ). By contrast, Ncr1 iCre/+ Ptpn6 flx/flx LAK cells were unable to secrete IFN-γ in the presence of YAC tumour cells ( Fig. 4b ). In addition, the ability of LAK cells from Ncr1 iCre/+ Ptpn6 flx/flx mice to kill YAC, RMA-S and RMA-Rae1 tumour cells in vitro was profoundly compromised ( Fig. 4c ). Thus, an absence of SHP-1 from NK cells decreased their cytotoxic and cytokine effector activities in response to tumour cells in vitro . 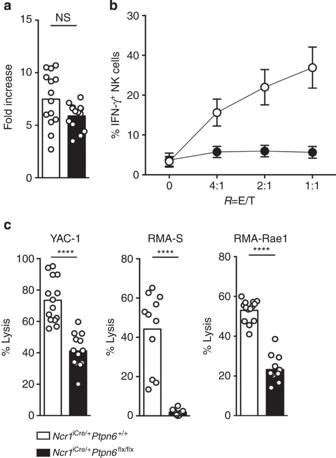Figure 4:In vitroNK cell hyporesponsiveness in the absence of SHP-1. (a) Fold-increase in NK cell numbers after 7 days of culture with IL-2 were obtained using a cell counter. (n=14,P=0.1164, Mann–Whitney). (b) Intracellular IFN-γ production by LAK cells on stimulation with YAC-1 tumour cells was measured by intracellular cytokine staining. (n=10,P<0.0001, two-way analysis of variance with Bonferroni correction). (c) LAK cell lysis of the YAC-1 (n=14), RMA-S (n=11) and RMA-Rae1 (n=4) cell lines measured in Cr51release assay. (P<0.0001, Mann–Whitney). Each dot on the histograms corresponds to the data from a single mouse (a,c) or the mean of several experiments (b); the data show the results of at least three independent experiments. Figure 4: In vitro NK cell hyporesponsiveness in the absence of SHP-1. ( a ) Fold-increase in NK cell numbers after 7 days of culture with IL-2 were obtained using a cell counter. ( n =14, P =0.1164, Mann–Whitney). ( b ) Intracellular IFN-γ production by LAK cells on stimulation with YAC-1 tumour cells was measured by intracellular cytokine staining. ( n =10, P <0.0001, two-way analysis of variance with Bonferroni correction). ( c ) LAK cell lysis of the YAC-1 ( n =14), RMA-S ( n =11) and RMA-Rae1 ( n =4) cell lines measured in Cr [51] release assay. ( P <0.0001, Mann–Whitney). Each dot on the histograms corresponds to the data from a single mouse ( a , c ) or the mean of several experiments ( b ); the data show the results of at least three independent experiments. Full size image Early signalling in NK cells in the absence of SHP-1 We then sought to dissect the mechanisms of the in vitro NK cell hyporeactivity in Ncr1 iCre/+ Ptpn6 flx/flx mice, by investigating the extent to which the absence of SHP-1 in NK cells controlled the early signalling events induced by the engagement of activating receptors. We focused on quantitative measurements of the two major signalling pathways: the generation of phosphatidylinositol trisphosphates (PtdIns(3,4,5) P 3 ) and intracytoplasmic Ca 2+ (iCa 2+ ) mobilization. The cytoplasmic membrane is composed of phosphatidylinositol phosphate (PtdIns(4) P ), bisphosphates (PtdIns(4,5) P 2 ) and a lower proportion of PtdIns(3,4,5) P 3 . Using a recently described highly sensitive mass spectrometry method [37] , we quantified the basal amounts of PtdIns(4) P , PtdIns(4,5) P 2 ( Supplementary Fig. 8 ) and the various molecular species of PtdIns(3,4,5) P 3 differing in terms of acyl chain composition (C18:0/C18:0, C18:0/C18:1, C18:0/C18:2, C18:0/C20:2, C18:0/C20:3 and C18:0/C20:4) ( Fig. 5a ). Ncr1 iCre/+ Ptpn6 +/+ and Ncr1 iCre/+ Ptpn6 flx/flx resting NK cells had similar basal levels of these different molecular species. Following their stimulation via Ly49D, control NK cells displayed a very early induction of C18:0/C20:3 and C18:0/C20:4 PtdIns(3,4,5) P 3 , 1 min after cross-linking, followed by a decline after 5 min of stimulation ( Fig. 5b ). The quantity, quality and kinetics of the PtdIns(3,4,5) P 3 generated did not differ significantly between NK cells isolated from Ncr1 iCre/+ Ptpn6 flx/flx mice and NK cells isolated from Ncr1 iCre/+ Ptpn6 +/+ mice ( Fig. 5a,b ). 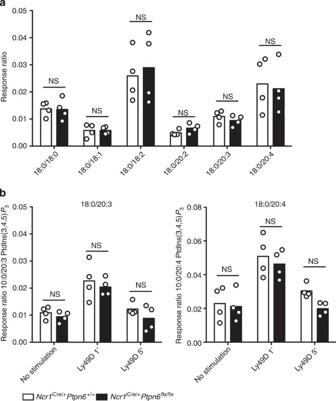Figure 5: Generation of PtdIns(3,4,5)P3molecular species induced by NK cell activation in the absence of SHP-1. (a) The basal amounts of the PtdIns(3,4,5)P3molecular species in the membrane of NK cells isolated fromNcr1iCre/+Ptpn6+/+andNcr1iCre/+Ptpn6flx/flxmice were determined by mass spectrometry. (n=4,P>0.9999, two-way analysis of variance (ANOVA) with Bonferroni correction.) (b) The amounts of C18:0/C20:3 and C18:0/C20:4 PtdIns(3,4,5)P3molecular species were determined after 1 (P>0.9999) or 5 min (18:0/20:3,P=0.7407 and 18:0/20:4,P=0.2894) of activation with anti-Ly49D mAbs cross-linked to with F(ab)’2 mAbs. The other molecular species of PtdIns(3,4,5)P3did not change significantly following stimulation. (n=4, two-way ANOVA with Bonferroni correction). Data are expressed as response ratio (integrated ion current response to the defined PtdIns(3,4,5)P3molecular species divided by that to the internal standard)45. Each dot on the histograms corresponds to the data for a NK cell preparation from a pool of four mice and the data show the results of two independent experiments. Figure 5: Generation of PtdIns(3,4,5) P 3 molecular species induced by NK cell activation in the absence of SHP-1. ( a ) The basal amounts of the PtdIns(3,4,5) P 3 molecular species in the membrane of NK cells isolated from Ncr1 iCre/+ Ptpn6 +/+ and Ncr1 iCre/+ Ptpn6 flx/flx mice were determined by mass spectrometry. ( n =4, P >0.9999, two-way analysis of variance (ANOVA) with Bonferroni correction.) ( b ) The amounts of C18:0/C20:3 and C18:0/C20:4 PtdIns(3,4,5) P 3 molecular species were determined after 1 ( P >0.9999) or 5 min (18:0/20:3, P =0.7407 and 18:0/20:4, P =0.2894) of activation with anti-Ly49D mAbs cross-linked to with F(ab)’2 mAbs. The other molecular species of PtdIns(3,4,5) P 3 did not change significantly following stimulation. ( n =4, two-way ANOVA with Bonferroni correction). Data are expressed as response ratio (integrated ion current response to the defined PtdIns(3,4,5) P 3 molecular species divided by that to the internal standard) [45] . Each dot on the histograms corresponds to the data for a NK cell preparation from a pool of four mice and the data show the results of two independent experiments. Full size image For the assessment of real-time iCa 2+ mobilization, freshly isolated NK cells from Ncr1 iCre/+ Ptpn6 flx/flx and Ncr1 iCre/+ Ptpn6 +/+ control mice were incubated in vitro with biotinylated monoclonal antibodies (mAbs) against Ly49D or NKG2D. Antibody-coated NK cells were then incubated with streptavidin for the assessment of real-time iCa 2+ mobilization by flow cytometry. Receptor-mediated iCa 2+ mobilization was assessed by determining the intensity of the [iCa 2+ ] peak and the integration of [iCa 2+ ] over time. As expected, binding to Ly49D or NKG2D led to an increase in [iCa 2+ ] in NK cells from Ncr1 iCre/+ Ptpn6 +/+ control mice ( Fig. 6a ). However, the peak of [iCa 2+ ] induced by Ly49D cross-linking was ~40% lower in NK cells from Ncr1 iCre/+ Ptpn6 flx/flx mice than in NK cells from Ncr1 iCre/+ Ptpn6 +/+ mice ( Fig. 6a (upper panel) and b). Moreover, iCa 2+ mobilization in the NK cells of Ncr1 iCre/+ Ptpn6 flx/flx mice was 90% weaker after incubation with NKG2D mAbs ( Fig. 6a (lower panel) and Fig. 6b ). Similar results were obtained with β2m −/− ( Supplementary Fig. 9a,b ) and, in both types of mice, no difference in iCa 2+ mobilization was observed when NK cells were stimulated with ionomycin ( Supplementary Fig. 9c ). Thus, the hyporeactivity of NK cells intrinsically lacking SHP-1 primarily affects iCa 2+ mobilization, but not generation of the second messenger PtdIns(3,4,5) P 3 induced by engagement of activating receptors. 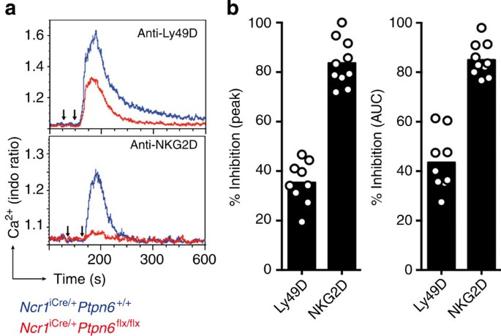Figure 6: iCa2+mobilization induced by NK cell activation in the absence of SHP-1. (a) iCa2+mobilization in freshly isolated NK cells, measured by flow cytometry.Ncr1iCre/+Ptpn6+/+(blue curve) andNcr1iCre/+Ptpn6flx/flx(red curve) NK cells were activated by incubation with biotinylated anti-Ly49D mAbs (first arrow, above) or biotinylated anti-NKG2D mAbs (first arrow, below), which were cross-linked with streptavidin 30 s later (second arrow). (b) Peak iCa2+mobilization and the area under the curve (AUC) are indicated as a % inhibition inNcr1iCre/+Ptpn6flx/flxNK cells with respect toNcr1iCre/+Ptpn6+/+NK cells. (Ly49D,n=9; NKG2D,n=10). Each dot on the histograms corresponds to the data for a NK cell preparation from a pool of four mice and the data show the results of three independent experiments. Figure 6: iCa 2+ mobilization induced by NK cell activation in the absence of SHP-1. ( a ) iCa 2+ mobilization in freshly isolated NK cells, measured by flow cytometry. Ncr1 iCre/+ Ptpn6 +/+ (blue curve) and Ncr1 iCre/+ Ptpn6 flx/flx (red curve) NK cells were activated by incubation with biotinylated anti-Ly49D mAbs (first arrow, above) or biotinylated anti-NKG2D mAbs (first arrow, below), which were cross-linked with streptavidin 30 s later (second arrow). ( b ) Peak iCa 2+ mobilization and the area under the curve (AUC) are indicated as a % inhibition in Ncr1 iCre/+ Ptpn6 flx/flx NK cells with respect to Ncr1 iCre/+ Ptpn6 +/+ NK cells. (Ly49D, n =9; NKG2D, n =10). Each dot on the histograms corresponds to the data for a NK cell preparation from a pool of four mice and the data show the results of three independent experiments. Full size image SHP-1 is a major mediator of MHC class I receptors inhibition Given the role of inhibitory MHC class I-specific receptors in NK cell tuning and the putative role of SHP-1 as an effector acting downstream from these inhibitory receptors, we assessed the impact of the lack of SHP-1 on the function of the MHC class I-specific receptors expressed on NK cells. The percentages of NK cells expressing inhibitory Ly49 receptors differed between Ncr1 iCre/+ Ptpn6 flx/flx and Ncr1 iCre/+ Ptpn6 +/+ mice ( Fig. 3a ). We therefore first focused on inhibitory CD94/NKG2A heterodimers and activating Ly49D receptors, the expression of which was not affected by the lack of SHP-1 in NK cells ( Fig. 3b ). The inhibitory function of ITIM-bearing molecules is dependent on their co-aggregation with activating receptors [21] . In NK cells, only activating receptors stimulated together with MHC class I-specific inhibitory receptors are affected, displaying lower levels of activation, whereas other activating receptors not co-engaged with inhibitory receptors are unaffected [21] . Freshly isolated NK cells from Ncr1 iCre/+ Ptpn6 flx/flx and Ncr1 iCre/+ Ptpn6 +/+ control mice were thus incubated in vitro with biotinylated Ly49D mAbs in the presence or absence of biotinylated NKG2A mAbs, and real-time iCa 2+ mobilization was measured. In Ncr1 iCre/+ Ptpn6 +/+ control mice, binding to Ly49D led to an increase in [iCa 2+ ], which was ~40% smaller if the CD94/NKG2A molecules were co-engaged ( Fig. 7a (upper panel) and b ). By contrast, almost no inhibition of Ly49D-induced iCa 2+ fluxes was observed when CD94/NKG2A molecules were co-engaged in Ncr1 iCre/+ Ptpn6 flx/flx mice ( Fig. 7a (lower panel) and b ). The co-engagement of NKG2A and Ly49D impaired Ly49D-induced iCa 2+ mobilization in NK cells isolated from β2m −/− mice, ruling out the possibility that the lack of inhibition of CD94/NKG2A heterodimers in Ncr1 iCre/+ Ptpn6 flx/flx NK cells was due to their hyporeactivity ( Supplementary Fig. 10 ). 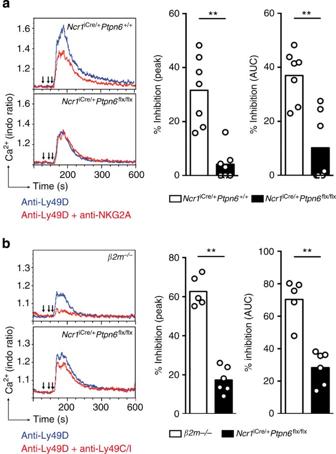Figure 7: SHP-1 is a major mediator of the inhibitory function of MHC class I-specific receptors. (a) iCa2+mobilization in freshly isolated NK cells fromNcr1iCre/+Ptpn6+/+mice (above) orNcr1iCre/+Ptpn6flx/flxmice (below). Blue curve: NK cells were treated with biotinylated anti-Ly49D mAbs (second arrow). Red curve: other NK cell preparations were treated with biotinylated anti-NKG2A mAbs (first arrow) and then with biotinylated anti-Ly49D mAbs (second arrow). Biotinylated antibodies were cross-linked with streptavidin (third arrow). (b) Peak iCa2+mobilization and the AUC for the indicated mice are indicated as a % inhibition for NK cells stimulated via Ly49D and NKG2A with respect to NK cells stimulated via Ly49D alone. (n=7, AUCP=0.0041 and peakP=0.0012, Mann–Whitney). (c) As ina, except that we used NK cells from β2m−/−(upper panel) mice orNcr1iCre/+Ptpn6flx/flxmice (lower panel), and these cells were stimulated via Ly49D (blue curve) or Ly49D and Ly49C/I (red curve). (d) Peak iCa2+mobilization and the AUC for the indicated mice are indicated as a % inhibition for NK cells stimulated via Ly49D and Ly49C/I with respect to NK cells stimulated via Ly49D alone. (β2 m−/−,n=5;Ncr1iCre/+Ptpn6flx/flx,n=6; AUC and peakP=0.0043, Mann–Whitney). Each dot on the histograms corresponds to the data for a NK cell preparation from a pool of four mice and the data the data show the results of two (c,d) or three (a,b) independent experiments. Figure 7: SHP-1 is a major mediator of the inhibitory function of MHC class I-specific receptors. ( a ) iCa 2+ mobilization in freshly isolated NK cells from Ncr1 iCre/+ Ptpn6 +/+ mice (above) or Ncr1 iCre/+ Ptpn6 flx/flx mice (below). Blue curve: NK cells were treated with biotinylated anti-Ly49D mAbs (second arrow). Red curve: other NK cell preparations were treated with biotinylated anti-NKG2A mAbs (first arrow) and then with biotinylated anti-Ly49D mAbs (second arrow). Biotinylated antibodies were cross-linked with streptavidin (third arrow). ( b ) Peak iCa 2+ mobilization and the AUC for the indicated mice are indicated as a % inhibition for NK cells stimulated via Ly49D and NKG2A with respect to NK cells stimulated via Ly49D alone. ( n =7, AUC P =0.0041 and peak P =0.0012, Mann–Whitney). ( c ) As in a , except that we used NK cells from β2m −/− (upper panel) mice or Ncr1 iCre/+ Ptpn6 flx/flx mice (lower panel), and these cells were stimulated via Ly49D (blue curve) or Ly49D and Ly49C/I (red curve). ( d ) Peak iCa 2+ mobilization and the AUC for the indicated mice are indicated as a % inhibition for NK cells stimulated via Ly49D and Ly49C/I with respect to NK cells stimulated via Ly49D alone. (β2 m −/− , n =5; Ncr1 iCre/+ Ptpn6 flx/flx , n =6; AUC and peak P =0.0043, Mann–Whitney). Each dot on the histograms corresponds to the data for a NK cell preparation from a pool of four mice and the data the data show the results of two ( c , d ) or three ( a , b ) independent experiments. Full size image For precise quantification of the inhibitory function of H-2K b -specific Ly49C/I molecules in the absence of SHP-1, we compared NK cells isolated from β2m −/− mice and Ncr1 iCre/+ Ptpn6 flx/flx mice, as these two types of mice had similar Ly49C/I cell percentages ( Fig. 3a and Supplementary Fig. 7a ). In β2m −/− mice, Ly49C/I inhibited Ly49D-mediated iCa 2+ mobilization by ~65% ( Fig. 7c (upper panel) and Fig. 7d ), consistent with the high percentage of Ly49C/I cells in these mice. By contrast, the inhibitory function of Ly49C/I was strongly impaired in Ncr1 iCre/+ Ptpn6 flx/flx mice ( Fig. 7c (lower panel) and Fig. 7d ). Thus, the absence of SHP-1 from NK cells impaired the inhibition mediated by Ly49C/I and CD94/NKG2A heterodimers, identifying SHP-1 as a major mediator of their inhibitory function in mouse NK cells. In vivo NK cell hyporesponsiveness in the absence of SHP-1 We then analysed the in vivo consequences of the in vitro hyporeactivity of NK cells lacking SHP-1. Control and Ncr1 iCre/+ Ptpn6 flx/flx mice received injections of a 1:1 mixture of wild-type and β2m −/− splenocytes, in a standard in vivo missing-self-recognition assay [13] , [38] , [39] . As expected, control mice rejected β2m −/− splenocytes ( Fig. 8a ) due to the lack of engagement of inhibitory MHC class I receptors on recipient NK cells by β2m −/− splenocytes. By contrast, Ncr1 iCre/+ Ptpn6 flx/flx mice were unable to reject β2m −/− splenocytes ( Fig. 8a ). Thus, NK cells from Ncr1 iCre/+ Ptpn6 flx/flx mice cannot eliminate MHC class I-deficient cells in vivo . 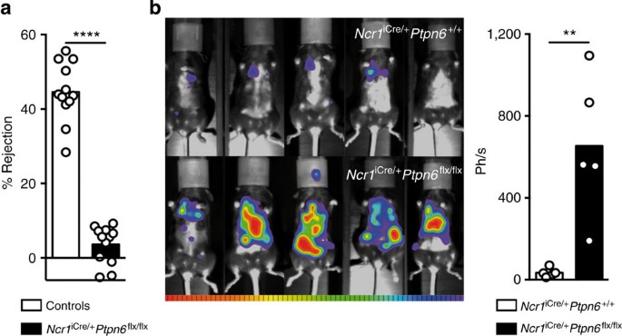Figure 8:In vivoNK cell hyporesponsiveness in the absence of SHP-1. (a) Rejection of β2m−/−splenocytes by control mice (Ncr1iCre/+Ptpn6+/+orNcr1+/+Ptpn6flx/flx) andNcr1iCre/+Ptpn6flx/flxmice, 20 h after their intravenous (i.v.) injection. Each dot on the histograms corresponds to the data for a single mouse and the data show the results of four independent experiments. (n=12,P<0.0001, Mann–Whitney). (b) Bioluminescence imaging ofNcr1iCre/+Ptpn6+/+(top) andNcr1iCre/+Ptpn6flx/flx(bottom) mice, 16 days after the i.v. injection of luciferase+B16-melanoma cells. On the right, quantification in photons per second of the bioluminescence from B16-melanoma cells 16 days after i.v. injection (n=5,P=0.0079, Mann–Whitney). Each dot on the histograms corresponds to the data for a single mouse. Figure 8: In vivo NK cell hyporesponsiveness in the absence of SHP-1. ( a ) Rejection of β2m −/− splenocytes by control mice ( Ncr1 iCre/+ Ptpn6 +/+ or Ncr1 +/+ Ptpn6 flx/flx ) and Ncr1 iCre/+ Ptpn6 flx/flx mice, 20 h after their intravenous (i.v.) injection. Each dot on the histograms corresponds to the data for a single mouse and the data show the results of four independent experiments. ( n =12, P <0.0001, Mann–Whitney). ( b ) Bioluminescence imaging of Ncr1 iCre/+ Ptpn6 +/+ (top) and Ncr1 iCre/+ Ptpn6 flx/flx (bottom) mice, 16 days after the i.v. injection of luciferase + B16-melanoma cells. On the right, quantification in photons per second of the bioluminescence from B16-melanoma cells 16 days after i.v. injection ( n =5, P =0.0079, Mann–Whitney). Each dot on the histograms corresponds to the data for a single mouse. Full size image We also injected luciferase + B16 melanoma cells intravenously into Ncr1 iCre/+ Ptpn6 flx/flx or control Ncr1 iCre/+ Ptpn6 +/+ mice and assessed tumour growth over time by bioluminescence imaging. The development of B16 melanoma cells in vivo is known to be controlled by NK cells ( Supplementary Fig. 11 ) [40] . By contrast to what was observed for Ncr1 iCre/+ Ptpn6 +/+ mice, massive B16 tumour development was observed in Ncr1 iCre/+ Ptpn6 flx/flx mice ( Fig. 8b ). Ncr1 iCre/+ Ptpn6 flx/flx NK cells thus display a marked hyporeactivity in vivo , characterized by their inability to reject MHC class I-deficient haematopoietic cells and B16 melanoma tumours. We describe here the impact of an intrinsic lack of SHP-1 in mouse NK cells. Unlike other immune cells, such as B cells [30] , CD4 + T cells [41] , regulatory T cells [42] , dendritic cells and neutrophils [43] , we show here that SHP-1-deficient NK cells are hyporesponsive and do not promote inflammation or autoimmunity. NK cells are, to our knowledge, the only cell type in which a lack of SHP-1 increases, rather than decreases, the activation threshold. Indeed, we show that SHP-1 expression in NK cells is required for their functional competence. In the absence of SHP-1, NK cells were present, but their phenotype resembled that of NK cells from MHC class I-deficient hosts, with impaired KLRG-1 expression, a skewing of the repertoire of inhibitory Ly49 receptors and a hyporesponsiveness of NK cells to various tumours and to MΗC class I-negative haematopoietic grafts. Ly49 knockdown mice (NKC KD ) also present some of these features, as they are also hyporesponsive in vivo to MΗC class I-negative haematopoietic grafts and tumours [18] . Many receptors and pathways are regulated by SHP-1 in lymphocytes, including NK cells [44] . The similarity of the phenotypes associated with an absence of SHP-1 and an absence of MHC class I receptor engagement strongly suggests that SHP-1 is used principally by Ly49 and NKG2A in NK cells. Our findings are consistent with the NK cell hyporesponsiveness induced by the transdominant negative form of SHP-1, although the alteration in NK cell function was less pronounced, probably due to the partial impairment of SHP-1 function in this experimental model [27] . A paradox thus remains to be resolved: how can the lack of a protein tyrosine phosphatase that downregulates NK cell activation when recruited by inhibitory receptors lead to NK cell hyporesponsiveness rather than hyperactivation, as in other lymphocytes? Our dissection of the mechanisms underlying NK cell tuning by MHC class I receptors was based on two aspects. First, in the absence of SHP-1, the inhibitory function of MHC class I receptors (CD94/NKG2A heterodimers and Ly49C/I receptors) was barely detectable. Thus, although ITIM-bearing MHC class I receptors can bind SHP-2 (refs 21 , 22 ) or be linked to Crk phosphorylation [24] , our data indicate that SHP-1 is a key signalling molecule for the inhibitory function of MHC class I receptors in mouse NK cells. These findings are consistent with those for the silencing of Ptpn6 , which results in an inability of ITIM-bearing inhibitory receptors to prevent the activation of mouse primary NK cells [45] . Second, we found that the intrinsic lack of inhibitory MHC class I receptor function was linked to NK cell hyporesponsiveness. Thus, our data are consistent with a model in which, in the absence of MHC class I detection, NK cells are desensitized due to their unrestrained activation by the chronic recognition of endogenous stimulating ligands in vivo , that is, the disarming model [14] . The induction of cell desensitization by the sustained activation of signalling elements is a very common mechanism that has been conserved throughout evolution. NK cells are innate lymphocytes expressing a wide panel of activating receptors, cytokine receptors and adhesion molecules [2] . Some of the ligands of these activating receptors are induced by various forms of cellular stress, ranging from microbial infection to tumour transformation, but other ligands are expressed constitutively in steady-state conditions in healthy organisms. This is the case for adhesion molecules, SLAM-family members, Nectin-like molecules and cytokines, such as IL-15 (refs 46 , 47 ). Thus, NK cells can respond to many endogenous ligands, at all stages of development. This high likelihood of NK cell activation by endogenous ligands contrasts with that of T and B cells, which is much lower due to a combination of the clonal organization of their responses and the selection and specificity of their antigen receptor repertoires. Our model of NK cell desensitization is supported by previous studies, in which the chronic expression of ligands for activating NK cell receptors was found to lead to NK cell hyporesponsiveness in vitro and in vivo [48] , [49] , [50] , [51] . It has also been described in humans, for NK cells expressing the activating KIR2S1 receptors in individuals bearing the cognate HLA-C2 group molecules [52] . As an alternative to the model of NK cell desensitization, it could be proposed that the lack of inhibition results in a developmental block yielding CD11b + CD27 + NK cells that, in an attempt to acquire an inhibitory receptor, continue to accumulate inhibitory Ly49 receptor at their surface [14] . We do not favour this possibility as Ncr1 iCre/+ Ptpn6 flx/flx NK cells present only a moderate change in their maturation profile as judged by the cell surface expression of CD11b and CD27; however, further experiments would be required to fully exclude this possibility. Which signalling components are affected by the sustained absence of SHP-1 activity in NK cells and which are involved in NK cell hyporesponsiveness? We focused our analysis on the signalling elements known to be targeted by SHP-1 and on the NKG2D- and Ly49D-dependent signalling pathways, which we showed to be impaired in SHP-1-deficient NK cells. SHP-1 can downregulate the activation of many signalling molecules, including Src family protein tyrosine kinases (SFKs), Vav1, SLP-76, phosphoinositide phospholipase C-γ (PLC-γ) and phosphoinositide 3-kinase (PI3K) [22] , [44] , [53] . In resting mouse NK cells, NKG2D associates with DAP10 (ref. 54 ), triggering two signalling pathways. DAP10 activates a Grb2, Vav1, SLP-76 signalosome, which in turn activates PLC-γ, leading to iCa 2+ mobilization. It also activates PI3K [55] , leading to the generation of PtdIns(3,4,5) P 3 from PtdIns(4,5) P 2 . Ly49D associates with the ITAM-bearing polypeptide DAP12, providing a link to the PLC-γ and PI3K pathways [53] . Both iCa 2+ mobilization and PtdIns(3,4,5) P 3 metabolites are essential for NK cell effector function [22] , [53] , [56] . We observed no major effect of the lack of SHP-1 on the generation of different molecular species of PtdIns(3,4,5) P 3 induced by NK cell activation, indicating that changes to the PI3K pathway play no major role in the NK cell hyporesponsiveness observed in Ncr1 iCre/+ Ptpn6 flx/flx mice. By contrast, there are several lines of evidence to suggest that an intrinsic lack of SHP-1 in NK cells might lead to the impairment of other protein tyrosine kinase-dependent pathways. Indeed, SHP-1 can control the activation of SFK members [44] . In addition, formation of the Ly49 repertoire is dependent on the activity of the SFK member Fyn [57] . As we show here that the absence of SHP-1 leads to an impairment of iCa 2+ mobilization on Ly49D or NKG2D engagement, the model that best fits our data is the desensitization of NK cells in the absence of SHP-1, in a process involving sustained protein tyrosine kinase-dependent activation. The duration of exposure of NK cells to endogenous signals likely to trigger their desensitization is a key factor. The formal demonstration of the involvement of Fyn, Vav1, SLP-76 or PLC-γ in this process will thus require the generation of inducible models of NK cell-specific gene deletions, such as NKp46-iCre/ER knock-in mice. Regardless of the results obtained in such experiments, the role of SHP-1 in NK cell education described here is consistent with our previous findings that the confinement of activating receptors to the plasma membrane plays a key role in ensuring the self-tolerance of NK cells [36] . Indeed, it is possible that in the absence of inhibition mediated by MHC class I receptors, activating receptors engaged due to frequent encounters with endogenous ligands might migrate to the actin meshwork within the membrane, thereby contributing to the hyporesponsiveness of NK cells. Thus, our data support a model in which SHP-1 is required for the maintenance of a functional NK cell repertoire. SHP-1-expressing NK cells are functionally competent in terms of their activation receptors. By contrast, SHP-1-deficient NK cells have no functional self-MHC class I-specific inhibitory receptors and are hyporeactive. However, in both situations NK cells are self-tolerant. SHP-1-expressing NK cells are tolerant because they have functional inhibitory receptors for self-MHC class I, and SHP-1-deficient NK cells are tolerant because of their hyporesponsiveness. To the best of our knowledge, the description of this adaptive response of NK cells involving SHP-1 constitutes the first report of an immune tolerance strategy of this type. Mice Ncr1 iCre/+ mice have been described elsewhere [10] . Ptpn6 flx/flx mice were obtained from the Jackson Laboratory. Ptpn6 is located on mouse chromosome 6, close to the NK gene ( Nkc ) complex. We therefore backcrossed Ncr1 iCre/+ Ptpn6 flx/flx mice to obtain recombinant animals with an Nkc complex of C57/BL/6 origin, as demonstrated by the cell surface expression of NK1.1 on NK cells from Ncr1 iCre/+ Ptpn6 flx/flx mice. Mice were bred and maintained under specific pathogen-free conditions at the Centre d’explorations physio-pathologiques avancées in Marseilles. Female and male mice of 6–12 weeks were used for the experiments. Mice were maintained in specific pathogen-free conditions and all experiments were done in accordance with institutional committees and French and European guidelines for animal care. Cell preparation Splenocyte suspensions were obtained by the mechanical disruption of mouse spleen, and blood cells were then lysed in RBC lysis solution (eBioscience). Splenocytes were used for NK cell marker analyses, in vitro experiments concerning NK cell activation and enriched NK cell production. Preparations enriched in NK cells with the NK Cell Isolation Kit II (Miltenyi Biotec) were used for Ca 2+ flux and PtdIns(3,4,5) P 3 determinations and for LAK cell production. LAK cells were obtained after 7 days of culture with IL-2 (5,000 U ml −1 , Chiron). LAK cells were used for SHP-1 western blottings and in vitro experiments. Cell purity, assessed by flow cytometry, was 70–80% for cell preparations enriched in NK cells and 95–99% for LAK cells. Mice were anaesthetized and immediately perfused with PBS before the collection of the liver and gut. Livers were mechanically disrupted in PBS, in a cell strainer, and the cell suspensions were washed three times with PBS. Samples were then enriched in lymphocytes by centrifugation on a Percoll gradient (GE Healthcare). Cells from the small intestine were prepared as previously described [58] . In brief, 2- to 3-cm intestine pieces were washed three times with PBS 1 × and then incubated at 37 °C during 15 min in 20 ml of PBS 1 × , HEPES 1 M, EDTA 0.5 M and FCS 10% before a final wash in RPMI 10% FCS. The tissues were then incubated three times at 37 °C during 15 min in 20 ml of RPMI, 10% FCS, HEPES 1 M and collagenase VIII (Sigma) 300 UI ml −1 . At each round of digestion, intestinal cells were harvested in the supernatant, washed in RPMI, 10% FCS and enriched in lymphocytes by centrifugation on Percoll gradient. Blood cell counts were quantified by flow cytometry using Trucount tubes (BD Biosciences). Flow cytometry Flow cytometry analysis was performed on a BD LSR II (four laser Blue/Red/Violet/utraviolet flow cytometry analyser, BD Biosciences). Antibodies against RORγt-PE (AFKJS-9 1/50), NKp46-PreCP (29A1.4 1/100), CD49d-PE (DX5 1/400), CD49a-APC (Ha31/8 1/400), CD27-PE (LG.3A10 1/100), CD11b-V450 (M1/70 1/600), Ly49G2-PC7 (4D11 1/400), Ly49A-V450 (Ye1/48.10.6 1/400), Ly49F-PE (HBF-719 1/200), Ly49C/I-biot (5E6), Ly49H-APC (3D10 1/400), Ly49D-FITC (4E5 1/800), NKG2A-biot (16a11 1/100), NKG2D-PE (Cx5 1/50), KLRG1 (2F1 1/400), CD107a-FITC (1D4B 1/50) and IFN-γ-A647 (XMG1.2 1/200) NK1.1-PC7 (PK136 1/400) were obtained from eBioscience, Biolegend and BD Biosciences, and stained with LIVE/DEAD Fixable Dead Cell Stain (Molecular Probes). In vitro cell activation For the measurement of IFN-γ production, splenocytes were activated with cytokines (25 ng ml −1 IL-12 from eBioscience and 20 ng ml −1 IL-18 from MBL) or in 96-well plates coated with anti-NK1.1 antibody (30 μg ml −1 , eBioscience) or Ly49D (30 μg ml −1 , BD Biosciences). LAK cells were coincubated with YAC-1 cells in various ratios (effector/target): 4/1, 2/1 and 1/1. Cells were activated by incubation with monensin and brefeldin A (GolgiPlug and GolgiStop BD) in complete medium for 4 h at 37 °C. The cells were subjected to surface staining, then fixed with 1% paraformaldehyde and permeabilized with Perm/Wash solution (BD Biosciences) before IFN-γ staining. Cytotoxicity assays were performed with LAK cells coincubated for 4 h at 37 °C with target cell lines (YAC-1, RMA and RMA-Rae1, at a ratio of 10/1) preloaded with 51 Cr. The chromium released into culture supernatants was quantified in LumaPlate TopCount NXT microplate scintillation (Perkin Elmer). Ca 2+ mobilization Preparations enriched in NK cells were loaded by incubation for 1 h at 37 °C with Indo-1/AM (5 μM final concentration, Calbiochem) in Hank’s balanced salt solution (with Ca 2+ and Mg 2+ , without phenol red, PAA). Cells were washed and stained with anti-CD3-FITC and anti-NKp46-Alexa660 antibodies. Before acquisition, each tube (10 6 cells per ml) was warmed at 37 °C for 10 min. NK cells were activated with biotin-conjugated antibodies against NKG2D (eBioscience) or Ly49D (eBioscience). Thirty seconds before Ly49D activation, NK cells are inhibited or not with biotin-conjugated antibodies against NKG2A (eBioscience) or Ly49C/I (BD Biosciences). The antibodies were used at a final concentration of 2.5 μg ml −1 and were cross-linked with ImmunoPure streptavidin (10 μg ml −1 , Pierce), after 2 min of acquisition. Changes in intracellular Ca 2+ concentration over the time were monitored with the Indo-1 (violet) and Indo-1 (blue) channels on an LSR II UV flow cytometry analyser. Peak iCa 2+ mobilization and the area under the curve (AUC) are indicated as a % inhibition as follows: 100—( Ncr1 iCre/+ Ptpn6 flx/flx [peak or AUC] × 100/ Ncr1 iCre/+ Ptpn6 +/+ [peak or AUC] ). As positive controls of iCa 2+ mobilization, NK cells were activated with ionomycine (1 μg ml −1 , Sigma). Quantification of the phosphoinositides by mass spectrometry We stimulated one million cells of an NK cell-enriched preparation by incubation with an Ly49D antibody cross-linked to F(ab)’2 for 1 or 5 min, as indicated, in 170 μl of PBS containing 2 mM EDTA and 0.05% FCS. Reactions were stopped by adding 750 μl CHCl 3 /MeOH/1 M HCl (v/v/v: 10/20/1), phosphoinositides were extracted and PtdIns(3,4,5) P 3 molecular species were quantified by mass spectrometry [45] . Briefly, phosphoinositides were extracted with a two-phase system in which the lower organic phase contained lipids. The internal standard was added and phosphoinositides were derivatized by adding trimethylsilyl–diazomethane. The reaction was quenched by adding glacial acetic acid and phosphoinositides were extracted with the two-phase system. The organic phase was dried under an N 2 stream, resuspended in 100 μl of MeOH/H 2 O (v/v: 80/20) and subjected to mass spectrometry analysis by the lipidomics core facility of MetaToul and Inserm U1048-I2MC. Immunoblotting SHP-1 immunoblotting was performed with LAK cells. LAK cells were lysed with lysis buffer (25 mM HEPES, 150 mM NaCl, 1% NP40, 10 mM MgCl 2 , 1 mM EDTA, 2% glycerol and protease inhibitor cocktail tablets (Roche)). Protein assays were performed with a BCA kit (Pierce). We then subjected 10 μg of protein in LDS sample buffer (Invitrogen) to electrophoresis in a 4–12% Bis-Tris precast gel in MOPS SDS running buffer (Invitrogen). The bands obtained were transferred onto a nitrocellulose membrane with the iBlot Dry blotting system (Life Technologies). The membrane was saturated by incubation for 1 h with 0.5% Tween 20, 5% milk in PBS, stained with antibodies against SHP-1 (C-19, Santa Cruz) and then incubated with an anti-rabbit-horseradish peroxidase secondary antibody (Jackson Immunoresearch). Antibody binding was detected with an ECL kit (Amersham). After stripping, the same experiment is performed for β-actin revelation. β2m Rejection Splenocytes from β2m −/− mice were labelled with Dye eFluor 450 (10 μM, eBioscience) and splenocytes from wild-type mice were labelled with CFSE (3 μM, Life Technologies). In total, we mixed 10 × 10 6 cells of each population at a ratio of 1:1 and injected them intravenously into the mice. We harvested the spleens of the recipient mice 20 h later, and analysed the presence of labelled donor cells by flow cytometry. Percentage rejection=100−([(%β2m/%wt)output]/[(%β2m/%wt)input] × 100). B16-luciferase injection B16-luciferase melanoma cells were injected into the tail vein (3 × 10 5 per mouse). Luciferase expression was then monitored by bioluminescence imaging. We injected luciferin (OZ Biosciences) intraperitoneally into the mice (3 mg per mouse). After 15 min, the mice were anaesthetized and placed in a NightOwl LB981 in vivo Imager (Berthold Technologies). We used Berthold Technologies software to determine the number of photons emitted per second. Statistics Statistical significance was determined for Mann–Whitney tests and two-way analysis of variance with Bonferroni correction (Prism 5, GraphPad Software). The degree of significance is indicated as follows: * P <0.05, ** P <0.01, *** P <0.001 and **** P <0.0001. Sample size calculation was based on Student’s or analysis of variance statistics ( α =5%, 1− β (power)=80%, two-sided, to detect differences between groups ≧ 1.5 s.d.). According to these criteria, the minimum number of sample per group should be n =8. How to cite this article: Viant, C. et al. SHP-1-mediated inhibitory signals promote responsiveness and anti-tumour functions of natural killer cells. Nat. Commun. 5:5108 doi: 10.1038/ncomms6108 (2014).